On the existence of collective interactions reinforcing the metal-ligand bond in organometallic compounds 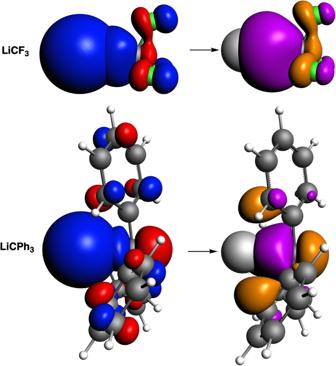Fig. 1: Overlap density between the two singly-occupied molecular orbitals (SOMOs) of LiCF3and LiCPh3. Isosurfaces of the superposed SOMO of Li• and the SOMO of •CR3(R = F, Ph) to construct LiCF3and LiCPh3(left, isovalue = 0.05 a.u.). Red and blue isosurfaces represent positive and negative phases. Overlap density between the two SOMOs (right, isovalue = 0.001 a.u.). Purple and orange isosurfaces indicate in-phase and out-of-phase overlap, respectively. See also Supplementary Figs.9–12. All calculations were performed with the Amsterdam Density Functional (ADF) module of the AMS2021 software package at the M06-2X/TZ2P level of theory [5] , [6] , [7] , [12] . The geometry optimizations were carried out without symmetry constraints (Supplementary Table 5 ). Numerical Hessians were computed to characterize the optimized structures as minima (zero imaginary frequencies). Geometries for LiCX 2 • and LiCX•• (X = F or Ph) were not allowed to relax but performed at the same geometry of LiCX 3 with the removal of either one (doublet state) or two X substituents (triplet state), respectively. LiCX 2 • and LiCX•• were computed at their doublet or triplet state, respectively. For this latter, the singlet state has been proven to be higher in energy in all cases. The Li–C interaction was analyzed within the framework of quantitative Kohn-Sham molecular orbital theory in combination with a quantitative activation strain model (ASM) and energy decomposition analysis (EDA) in the gas phase. Both homolytic and heterolytic breaking schemes of Li–C bond have been studied. For instance, in LiCF 3 , we may have Li• (one unpaired alpha electron) and •CF 3 (one unpaired beta electron) fragments for the homolytic breaking. Or we may have Li + and – CF 3 fragments in case of the heterolytic breaking. Activation strain and energy decomposition analysis For the activation strain model (ASM), the bond energy ∆ E between two fragments is made up of two components [3] , [13] : 
    E= E_strain+ E_int
 (1) Here, the strain energy ∆ E strain is the amount of energy required to deform the fragments from their equilibrium structure to the geometry that they acquire in the overall complex. The interaction energy ∆ E int corresponds to the actual energy change when the geometrically deformed fragments are combined to form the overall complex. We further analyze the interaction ∆ E int in the framework of the Kohn-Sham molecular orbital (MO) model, by dissecting it through our canonical energy decomposition analyses (EDA) into the electrostatic attraction, the Pauli repulsion and the (attractive) orbital interactions: 
    E_int= V_elstat+ E_Pauli+ E_oi
 (2) The term ∆ V elstat corresponds to the classical electrostatic interaction between the unperturbed charge distributions of the fragments in the geometry they possess in the complex. This term is usually attractive. The Pauli repulsion ∆ E Pauli between these fragments comprises the destabilizing interactions, associated with the Pauli principle for fermions, between occupied orbitals and is responsible for the steric repulsion. The orbital interaction ∆ E oi between these fragments in any MO model, and therefore also in Kohn-Sham theory, accounts for electron-pair bonding (the SOMO–SOMO interaction), charge transfer (empty/occupied orbital mixing between different fragments), and polarization (empty/occupied orbital mixing on one fragment due to the presence of another fragment). The orbital interaction energy ∆ E oi can be further decomposed into the contributions from each irreducible representation Γ of the interacting system. The use of M06-2X gives a term that cannot be decomposed, which is a correction term, such that the total orbital interaction is the correct one. Voronoi deformation density (VDD) charge The electron density distribution is analyzed by using the Voronoi deformation density (VDD) method for atomic charges [14] . The VDD atomic charge \({Q}_{{{{{\rm{A}}}}}}^{{{{{\rm{VDD}}}}}}\) is computed as the (numerical) integral of the deformation density Δ ρ ( r ) = ρ ( r ) – ∑ B ρ B ( r ) in the volume of the Voronoi cell of atom A [Eq. ( 3 )]. The Voronoi cell of atom A is defined as the compartment of space bound by the bond midplanes on and perpendicular to all bond axes between nucleus A and its neighboring nuclei (cf. the Wigner-Seitz cells in crystals) [14] . Q_A^VDD=-∫_Voronoi cell of A[ρ(r)-∑_Bρ_B(r)]dr
 (3) In Eq. ( 3 ), ρ ( r ) is the electron density of the molecule and \({\sum }_{{{{{\rm{B}}}}}}{\rho }_{{{{{\rm{B}}}}}}({{{{{\bf{r}}}}}})\) the superposition of atomic densities ρ B of a fictitious promolecule without chemical interactions that is associated with the situation in which all atoms are neutral. The interpretation of the VDD charge \({Q}_{{{{{\rm{A}}}}}}^{{{{{\rm{VDD}}}}}}\) is rather straightforward and transparent. Instead of measuring the amount of charge associated with a particular atom A, \({Q}_{{{{{\rm{A}}}}}}^{{{{{\rm{VDD}}}}}}\) directly monitors how much charge flows, due to chemical interactions, out of ( \({Q}_{{{{{\rm{A}}}}}}^{{{{{\rm{VDD}}}}}}\, > \,0\) ) or into ( \({Q}_{{{{{\rm{A}}}}}}^{{{{{\rm{VDD}}}}}}\, < \,0\) ) the Voronoi cell of atom A, that is, the region of space that is closer to nucleus A than to any other nucleus. ETS-NOCV calculations The natural orbitals for chemical valence method (ETS-NOCV) have been computed at the same M06-2X/TZ2P level of theory. It allows one to visualize the alteration in the electronic structure of the interacting species, which is associated with bond formation. In particular, we have depicted the deformation densities, whose shapes provide a visualization of the associated pairwise orbital interactions [15] .